Highly regio- and enantioselective multiple oxy- and amino-functionalizations of alkenes by modular cascade biocatalysis New types of asymmetric functionalizations of alkenes are highly desirable for chemical synthesis. Here, we develop three novel types of regio- and enantioselective multiple oxy- and amino-functionalizations of terminal alkenes via cascade biocatalysis to produce chiral α-hydroxy acids, 1,2-amino alcohols and α-amino acids, respectively. Basic enzyme modules 1–4 are developed to convert alkenes to ( S )-1,2-diols, ( S )-1,2-diols to ( S )-α-hydroxyacids, ( S )-1,2-diols to ( S )-aminoalcohols and ( S )-α-hydroxyacids to ( S )-α-aminoacids, respectively. Engineering of enzyme modules 1 & 2, 1 & 3 and 1, 2 & 4 in Escherichia coli affords three biocatalysts over-expressing 4–8 enzymes for one-pot conversion of styrenes to the corresponding ( S )-α-hydroxyacids, ( S )-aminoalcohols and ( S )-α-aminoacids in high e.e. and high yields, respectively. The new types of asymmetric alkene functionalizations provide green, safe and useful alternatives to the chemical syntheses of these compounds. The modular approach for engineering multi-step cascade biocatalysis is useful for developing other new types of one-pot biotransformations for chemical synthesis. Alkenes are readily available and excellent starting materials for chemical synthesis. Asymmetric functionalization of alkenes is of great importance in the synthesis of enantiopure chemicals for pharmaceutical manufacturing. Thus far, many metal catalyses have been developed for this, including the well-known Sharpless epoxidation [1] , dihydroxylation [2] aminohydroxylation [3] , Jacobsen epoxidation [4] and palladium-catalysed asymmetric alkene functionalization [5] . On the other hand, enzyme catalyses could provide green alternatives due to the non-toxicity, high selectivity and mild reaction conditions [6] , [7] , [8] . A number of enzyme-catalysed asymmetric alkene functionalizations have been reported, such as the epoxidation with monooxygenase or peroxidase [9] , dihydroxylation with dioxygenase [10] , hydration with hydratase [11] , and more recently, cyclopropanation and aziridination with engineered P450 enzymes [12] , [13] , [14] . Despite of these achievements, the development of new types of reactions and catalysts for asymmetric alkene functionalizations is highly wanted and remains a significant challenge. An attractive way of developing new asymmetric transformation is to develop novel cascade (tandem) catalysis for performing multi-step reactions sequentially or concurrently in one pot [15] , [16] . Recently, asymmetric hydroxy arylation and allylation of terminal alkenes was reported by combining platinum-catalysed diboration and palladium-catalysed cross-coupling [17] in a sequential manner due to divergent reaction conditions of diboration and cross-coupling. In comparison with cascade chemocatalysis or cascade hybrid catalysis [18] , cascade biocatalysis is of advantages in combining multiple and complex reactions due to the natural compatibility and similar reaction condition of many enzymes [19] , [20] , [21] , [22] , [23] , [24] , in addition to the green features of enzyme catalysis. Over the years, many types of non-natural biocatalytic cascades have been developed [25] , [26] , [27] , [28] , [29] , [30] , [31] , [32] , [33] , [34] , [35] , [36] . Nevertheless, the epoxidation–hydrolysis cascade for asymmetric trans -dihydroxylation of alkenes [37] , [38] , [39] recently developed by us is the only known biocatalytic cascade for asymmetric functionalization of alkenes. Thus far, most of the reported cascade biocatalysis enables only two to three relatively simple enzymatic reactions. It is very challenging to engineer the efficient cascade system containing more than four enzymatic reactions. We have keen interest in developing new types of asymmetric alkene functionalizations and engineering enzyme cascade containing more than four enzymatic reactions. One-pot regio- and stereoselective multiple oxy- and amino-functionalizations of terminal alkenes to produce chiral α-hydroxy acids, 1,2-amino alcohols and α-amino acids, respectively, are designed as the target reactions ( Fig. 1a ). Enantiopure α-hydroxy acid [40] , 1,2-amino alcohol [41] and α-amino acid [42] are the three very important groups of chiral chemicals with broad applications in chiral pharmaceutical and asymmetric syntheses. The designed new transformations could provide green, safe and complementary alternatives to the toxic cyanide-based asymmetric synthesis of chiral α-hydroxy acid (via cyanohydrin) [43] and α-amino acid (Strecker reaction) [44] and the osmium-based asymmetric synthesis of chiral amino alcohols [3] , [45] . Herein, we report the development of the three new types of asymmetric functionalizations of terminal alkenes, the modular approach for engineering efficient cascade biocatalysis containing more than four concurrent reactions, and the simple and green syntheses of α-hydroxy acids, 1,2-amino alcohols and α-amino acids in high enantiomeric excess (e.e.) and high yield. 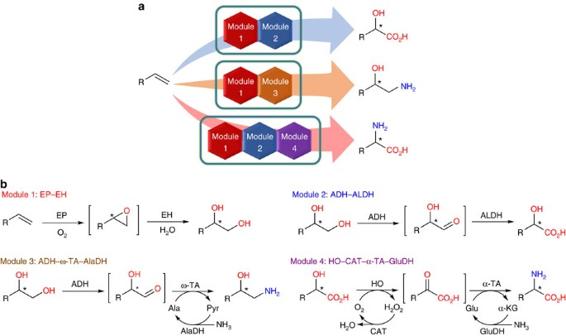Figure 1: Regio- and enantioselective multiple oxy- and amino-functionalizations of terminal alkenes by modular cascade biocatalysis. (a) One-pot conversion of terminal alkene to chiral α-hydroxy acid, 1,2-amino alcohol and α-amino acid withE. colicells containing multiple basic enzyme modules, respectively. (b) Four general basic enzyme modules and their cascade biotransformations. Module 1: epoxidase (EP) and epoxide hydrolase (EH) for epoxidation–hydrolysis of terminal alkene to 1,2-diol; Module 2: alcohol dehydrogenase (ADH) and aldehyde dehydrogenase (ALDH) for terminal double oxidation of 1,2-diol to α-hydroxy acid; Module 3: ADH, ω-transaminase (ω-TA) and alanine dehydrogenase (AlaDH) for oxidation–transamination of 1,2-diol to 1,2-amino alcohol; Module 4: hydroxy acid oxidase (HO), α-transaminase (α-TA), catalase (CAT) and glutamate dehydrogenase (GluDH) for oxidation–transamination of α-hydroxy acid to α-amino acid. Figure 1: Regio- and enantioselective multiple oxy- and amino-functionalizations of terminal alkenes by modular cascade biocatalysis. ( a ) One-pot conversion of terminal alkene to chiral α-hydroxy acid, 1,2-amino alcohol and α-amino acid with E. coli cells containing multiple basic enzyme modules, respectively. ( b ) Four general basic enzyme modules and their cascade biotransformations. Module 1: epoxidase (EP) and epoxide hydrolase (EH) for epoxidation–hydrolysis of terminal alkene to 1,2-diol; Module 2: alcohol dehydrogenase (ADH) and aldehyde dehydrogenase (ALDH) for terminal double oxidation of 1,2-diol to α-hydroxy acid; Module 3: ADH, ω-transaminase (ω-TA) and alanine dehydrogenase (AlaDH) for oxidation–transamination of 1,2-diol to 1,2-amino alcohol; Module 4: hydroxy acid oxidase (HO), α-transaminase (α-TA), catalase (CAT) and glutamate dehydrogenase (GluDH) for oxidation–transamination of α-hydroxy acid to α-amino acid. Full size image Design of modular biocatalysis for cascade reactions To realize the targeted asymmetric alkene functionalizations ( Fig. 1a ), we designed microbial cells containing two to three basic enzyme modules, each of them catalysing two to four enzymatic reactions ( Fig. 1b ), based on biocatalytic retrosynthesis analysis [46] . The basic modules were designed by using the following criteria: (a) each module utilizes a stable input, such as alkene, diol and hydroxy acid, and gives a stable output, such as diol, hydroxy acid, amino alcohol and amino acid; (b) each module enables fast conversion of unstable or toxic intermediates, such as epoxide, hydroxy aldehyde and keto acid, to minimize their accumulation and side reactions. Assemblies of module 1 and 2 in one cell, module 1 and 3 in one cell and module 1, 2 and 4 in one cell gave rise to whole-cell catalysts for one-pot transformations of terminal alkene to chiral α-hydroxy acid, 1,2-amino alcohol and α-amino acid, respectively ( Fig. 1a ). To demonstrate the concept, we chose the biotransformations of styrenes 1a–k to ( S )-α-hydroxy acids 5a–k , ( S )-1,2-amino alcohols 6a–k and ( S )-α-amino acids 8a–k , respectively, as the representative examples of the three types of asymmetric reactions ( Fig. 2 ). While the styrenes are easily available substrates, the ( S )-α-hydroxy acids, ( S )-1,2-amino alcohols and ( S )-α-amino acids are highly valuable chiral chemicals with many applications ( Supplementary Table 1 ). 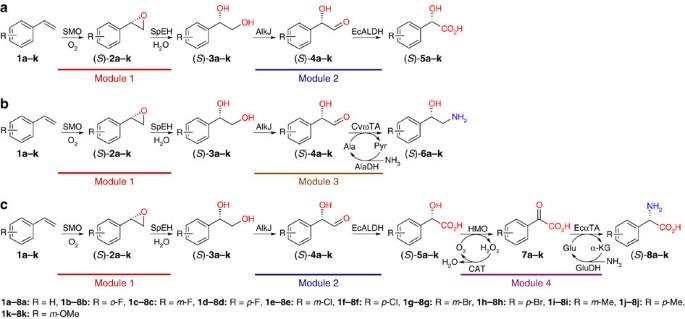Figure 2: Regio- and enantioselective multiple oxy- and amino-functionalizations of styrenes by modular cascade biocatalysis. (a) Conversion of styrenes to (S)-α-hydroxy acids withE. colistrains containing enzyme module 1 and 2. (b) Conversion of styrenes to (S)-1,2-amino alcohols withE. colistrains containing enzyme module 1 and 3. (c) Conversion of styrenes to (S)-α-amino acids withE. colistrains containing enzyme module 1, 2 and 4. SMO: styrene monooxygenase fromPseudomonassp. VLB120; SpEH: epoxide hydrolase fromSphingomonassp. HXN-200; AlkJ: alcohol dehydrogenase fromP. putidaGPo1; EcALDH: phenylacetaldehyde dehydrogenase fromE. coli; CvωTA: ω-transaminase fromC. violaceum; AlaDH: alanine dehydrogenase fromB. subtilis; HMO: hydroxymandelate oxidase fromS. coelicolorA3(2); EcαTA: branch chain amino acid transaminase fromE. coli; GluDH: glutamate dehydrogenase fromE. coli; and CAT: catalase fromE. coli. Figure 2: Regio- and enantioselective multiple oxy- and amino-functionalizations of styrenes by modular cascade biocatalysis. ( a ) Conversion of styrenes to ( S )-α-hydroxy acids with E. coli strains containing enzyme module 1 and 2. ( b ) Conversion of styrenes to ( S )-1,2-amino alcohols with E. coli strains containing enzyme module 1 and 3. ( c ) Conversion of styrenes to ( S )-α-amino acids with E. coli strains containing enzyme module 1, 2 and 4. SMO: styrene monooxygenase from Pseudomonas sp. VLB120; SpEH: epoxide hydrolase from Sphingomonas sp. HXN-200; AlkJ: alcohol dehydrogenase from P. putida GPo1; EcALDH: phenylacetaldehyde dehydrogenase from E. coli ; CvωTA: ω-transaminase from C. violaceum ; AlaDH: alanine dehydrogenase from B. subtilis ; HMO: hydroxymandelate oxidase from S. coelicolor A3(2); EcαTA: branch chain amino acid transaminase from E. coli ; GluDH: glutamate dehydrogenase from E. coli ; and CAT: catalase from E. coli . Full size image Engineering of basic enzyme modules Enzyme module 1 for the conversion of alkene to diol was engineered according to our previously reported method [39] . Escherichia coli (R-M1) containing gene module 1 on plasmid pRSFDuet-1 ( Table 1 ) was constructed to coexpress styrene monooxygenase (SMO) [47] and epoxide hydrolase (SpEH) [48] ( Fig. 2a ). As shown in Fig. 3a , 5 g cdw l –1 of E. coli (R-M1) cells efficiently transformed 50 mM styrene 1a to 46 mM ( S )-1-phenyl-1,2-ethanediol 3a in 5 h, without significant accumulation of ( S )-styrene oxide 2a (<1%). For further assembly of multiple basic modules and optimization of enzyme expression in one E. coli strain, gene module 1 was sub-cloned into other three different but compatible plasmids, pACYCDuet-1, pCDFDuet-1 and pETDuet-1, to generate three new recombinant plasmids, A-M1, C-M1 and E-M1, respectively ( Table 1 ). Table 1 Genetic construction of recombinant E. coli strains containing different enzyme modules. 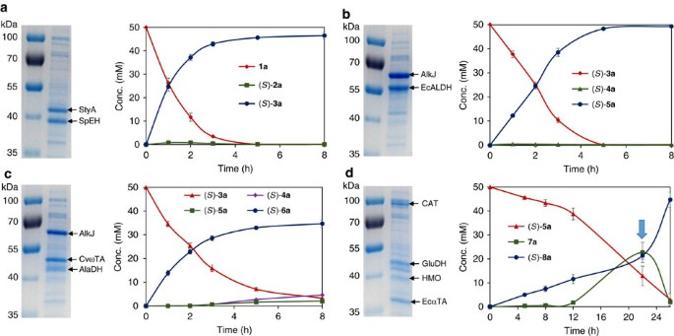Figure 3: SDS–PAGE and biotransformation time course ofE. colistrains containing individual enzyme modules. (a)E. coli(R-M1) cells containing enzyme module 1 (SMO and SpEH); and biotransformation of styrene1ato (S)-1-phenyl-1,2-ethanediol3a. (b)E. coli(R-M2) cells containing enzyme module 2 (AlkJ and EcALDH); and biotransformation of (S)-1-phenyl-1,2-ethanediol3ato (S)-mandelic acid5a. (c)E. coli(R-M3) cells containing enzyme module 3 (AlkJ, CvωTA and AlaDH); and biotransformation of (S)-1-phenyl-1,2-ethanediol3ato (S)-phenylethanolamine6a. (d)E. coli(R-M4) cells containing enzyme module 4 (HMO, EcαTA, GluDH and CAT); and biotransformation of (S)-mandelic acid5ato (S)-phenylglycine8a(blue arrow: adding additional 0.5% glucose at 22 h). All biotransformations were performed in triplicate, and error bars show±s.d. Full size table Figure 3: SDS–PAGE and biotransformation time course of E. coli strains containing individual enzyme modules. ( a ) E. coli (R-M1) cells containing enzyme module 1 (SMO and SpEH); and biotransformation of styrene 1a to ( S )-1-phenyl-1,2-ethanediol 3a . ( b ) E. coli (R-M2) cells containing enzyme module 2 (AlkJ and EcALDH); and biotransformation of ( S )-1-phenyl-1,2-ethanediol 3a to ( S )-mandelic acid 5a . ( c ) E. coli (R-M3) cells containing enzyme module 3 (AlkJ, CvωTA and AlaDH); and biotransformation of ( S )-1-phenyl-1,2-ethanediol 3a to ( S )-phenylethanolamine 6a . ( d ) E. coli (R-M4) cells containing enzyme module 4 (HMO, EcαTA, GluDH and CAT); and biotransformation of ( S )-mandelic acid 5a to ( S )-phenylglycine 8a (blue arrow: adding additional 0.5% glucose at 22 h). All biotransformations were performed in triplicate, and error bars show±s.d. Full size image To engineer enzyme module 2 for the conversion of diol to α-hydroxy acid, many commercially available alcohol dehydrogenases (ADH), cloned ADHs and wild-type strains collected in our laboratory ( Supplementary Table 2 ) were screened for the terminal oxidation of ( S )-1-phenyl-1,2-ethanediol 3a to identify a highly regioselective enzyme for the first reaction of the module ( Fig. 2a ). AlkJ from Pseudomonas putida GPo1 (ref. 49 ), a membrane-associated non-canonical ADH, was found to oxidize 3a at the terminal position to give mandelaldehyde 4a and mandelic acid 5a with S -enantioselectivity. Phenylacetaldehyde dehydrogenase (EcALDH, encoded by padA ) from E. coli [50] was then found to fully oxidize α-hydroxy aldehyde 4a to give 5a , the second reaction of the module. Thus, the genes of AlkJ and EcALDH were genetically engineered into a non-natural operon as gene module 2 on plasmid pRSFDuet-1 (R-M2, Table 1 ). E. coli (R-M2) cells expressed both AlkJ and EcALDH very well ( Fig. 3b ) and catalysed the highly regioselective terminal oxidation of 50 mM ( S )- 3a to give 49 mM ( S )- 5a in 8 h ( Fig. 3b ), without the accumulation of intermediate ( S )- 4a . Similarly, gene module 2 was also sub-cloned to the three plasmids to generate new recombinant plasmids, A-M2, C-M2 and E-M2, respectively ( Table 1 ). Enzyme module 3 is for the conversion of diol to α-amino alcohol. AlkJ-catalysed highly regioselective oxidation of ( S )- 3a to ( S )- 4a is the first reaction of module 3 ( Fig. 2b ). The ω-transaminase from Chromobacterium violaceum (CvωTA, encoded by cv_2025 ) [51] was chosen for the transamination of ( S )- 4a , the second reaction of the module. An E. coli strain was engineered to coexpress AlkJ and CvωTA and used for the biotransformation of 45 mM ( S )- 3a with 200 mM L -alanine as amine donor. While the desired product ( S )-phenylethanolamine 6a was produced (50% yield; 22 mM), some ( S )- 4a (14 mM) and ( S )- 5a (5 mM) remained in the system ( Supplementary Fig. 1 ). To increase the formation of ( S )- 6a in the reversible transamination reaction and utilize the cellular L -alanine and pyruvate, L -alanine dehydrogenase (AlaDH, encoded by ald , Genbank ID 936557) from Bacillus subtilis was used to regenerate L -alanine from cellular pyruvate with ammonia as amine donor [52] . A non-natural operon (gene module 3) containing the genes of AlkJ, CvωTA and AlaDH was cloned into the plasmid pRSFDuet-1 (R-M3, Table 1 ). The E. coli (R-M3) strain coexpressed the three enzymes well and catalysed the biotransformation of 50 mM ( S )- 3a to afford 35 mM ( S )- 6a in 8 h by using 200 mM ammonia with no addition of L -alanine ( Fig. 3c ). Substrate ( S )- 3a , intermediate ( S )- 4a , and by-product ( S )- 5a remained in relatively low amount (3, 5 and 2 mM, respectively). This in vivo amination with coexpressed ω-TA and AlaDH is complementary to the recently developed in vitro system [26] , [52] . Similarly, gene module 3 was sub-cloned into other three plasmids to generate A-M3, C-M3 and E-M3 ( Table 1 ). Enzyme module 4 is for the conversion of α-hydroxy acid to α-amino acid. To engineer this module, mandelate dehydrogenase [53] and hydroxymandelate oxidase (HMO, encoded by sco3228 ) from Streptomyces coelicolor A3(2) [54] were cloned into E. coli and examined for the oxidation of ( S )- 5a , respectively ( Fig. 2c ). HMO was found to be more efficient than the dehydrogenase ( Supplementary Fig. 2 ), thus being chosen as the first enzyme of module 4. For the enantioselective amination of 7a to ( S )- 8a , an amino acid dehydrogenase and four α-transaminases (α-TA) were screened with either ammonia or glutamate as amine donor ( Supplementary Fig. 3 ). EcαTA, the branch chain amino acid transaminase from E. coli (encoded by ilvE , Genbank ID 948278), was found to give the best results. Glutamate dehydrogenase (GluDH, encoded by gdhA , Genbank ID 946802) was then coexpressed with EcαTA in E. coli to enable the regeneration of glutamate by using ammonia during the transamination ( Supplementary Fig. 4 ). Since HMO is a H 2 O 2 -generating oxidase, a catalase (CAT, encoded by katE , Genbank ID 946234) was used to decompose H 2 O 2 to improve the biotransformation ( Supplementary Fig. 5 ). The genes of HMO, EcαTA, GluDH and CAT were thus engineered on plasmid pRSFDuet-1 (R-M4, Table 1 ) to construct module 4. E. coli (R-M4) coexpressed the four enzymes well ( Fig. 3d ) and converted 50 mM ( S )- 5a to 45 mM ( S )- 8a within 26 h ( Fig. 3d ). Gene module 4 was sub-cloned into three plasmids to give A-M4, C-M4 and E-M4, respectively ( Table 1 ). Engineering of catalyst to convert alkene to α-hydroxy acid Module 1 and 2 were assembled together in E. coli cells as the catalyst ( Fig. 2a ). To explore the optimal combination, four module 1 plasmids (A-M1, C-M1, E-M1 and R-M1) and four module 2 plasmids (A-M2, C-M2, E-M2 and R-M2) were combinatorially combined and transformed into E. coli . Since plasmids with the same backbone (for example, A-M1 and A-M2) are not compatible with each other, 12 E. coli strains were obtained ( Table 1 ), each co-expressing SMO, SpEH, AlkJ and EcALDH. These E. coli strains grew well in M9-glucose medium and expressed the desired enzymes. The collected cells were examined for the biotransformation of 100 mM styrene 1a in a two-liquid-phase system (buffer and n -hexadecane; 1:1) containing 0.5% glucose. As shown in Fig. 4a , all strains were able to convert 1a to ( S )- 5a (21–83 mM). Among them, three strains gave ( S )- 5a in 71–83 mM, and E. coli (A-M1_R-M2) is the best one to produce 83 mM ( S )- 5a (83% conversion) in 20 h together with 9 mM ( S )- 3a . SDS–PAGE analysis of the cell proteins of the 12 strains ( Supplementary Fig. 6 ) revealed that the three good strains exhibited a relatively balanced expression of the four enzymes, whereas several strains with lower productivity expressed much less AlkJ and EcALDH (module 2) than SMO and SpEH (module 1). The whole-cell activities of E. coli (A-M1_R-M2) towards 1a , ( S )- 2a , ( S )- 3a and ( S )- 4a were determined to be 43, 220, 29 and 42 U (g cdw) –1 , respectively. E. coli (A-M1_R-M2) was used to transform 100–150 mM 1a to ( S )- 5a , and the highest product concentration was observed with 120 mM 1a ( Supplementary Fig. 7a ). The time course of biotransformation of 120 mM 1a with 15 g cdw l –1 resting cells of E. coli (A-M1_R-M2) was shown in Fig. 4b . A total of 94 mM (14.2 g l –1 ) ( S )- 5a was produced in 98% e.e. and 78% conversion in 22 h. The unreacted substrate 1a and intermediate ( S )- 3a were found at a relatively low level (9 and 12 mM, respectively). 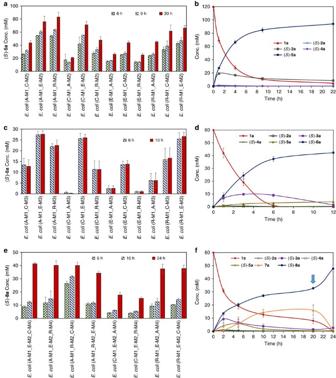Figure 4: Regio- and enantioselective multiple oxy- and amino-functionalizations of styrene 1a withE. colistrains containing multiple enzyme modules. (a) Product concentration of biotransformation of 100 mM1ato (S)-5awith twelveE. colistrains (10 g cdw l−1), each containing both enzyme module 1 and 2, respectively. (b) Time course of biotransformation of 120 mM1ato (S)-5awithE. coli(A-M1_R-M2) cells (15 g cdw l−1) in a two-liquid-phase system (KP buffer containing 0.25% glucose andn-hexadecane; 1:1) at 30 °C. (c) Product concentration of biotransformation of 50 mM1ato (S)-6awith twelveE. colistrains (10 g cdw l−1), each containing both enzyme module 1 and 3, respectively. (d) Time course of biotransformation of 60 mM1ato (S)-6awithE. coli(A-M1_E-M3) cells (15 g cdw l−1) in a two-liquid-phase system (NaP buffer containing 1% glucose and 200 mM NH3/NH4Cl andn-hexadecane; 1:1) at 25 °C. (e) Product concentration of biotransformation of 50 mM1ato (S)-8awith eightE. colistrains (10 g cdw l−1), each containing enzyme module 1, 2 and 4, respectively. (f) Time course of biotransformation of 60 mM1ato (S)-8awithE. coli(A-M1_R-M2_C-M4) cells (15 g cdw l−1) in a two-liquid-phase system (KP buffer containing 0.5% glucose and 100 mM NH3/NH4Cl andn-hexadecane; 1:1) at 30 °C (arrow: adding additional 0.5% glucose and 100 mM NH3/NH4Cl at 20 h). All biotransformations were performed in triplicate, and error bars show±s.d. Figure 4: Regio- and enantioselective multiple oxy- and amino-functionalizations of styrene 1a with E. coli strains containing multiple enzyme modules. ( a ) Product concentration of biotransformation of 100 mM 1a to ( S )- 5a with twelve E. coli strains (10 g cdw l −1 ), each containing both enzyme module 1 and 2, respectively. ( b ) Time course of biotransformation of 120 mM 1a to ( S )- 5a with E. coli (A-M1_R-M2) cells (15 g cdw l −1 ) in a two-liquid-phase system (KP buffer containing 0.25% glucose and n -hexadecane; 1:1) at 30 °C. ( c ) Product concentration of biotransformation of 50 mM 1a to ( S )- 6a with twelve E. coli strains (10 g cdw l −1 ), each containing both enzyme module 1 and 3, respectively. ( d ) Time course of biotransformation of 60 mM 1a to ( S )- 6a with E. coli (A-M1_E-M3) cells (15 g cdw l −1 ) in a two-liquid-phase system (NaP buffer containing 1% glucose and 200 mM NH 3 /NH 4 Cl and n -hexadecane; 1:1) at 25 °C. ( e ) Product concentration of biotransformation of 50 mM 1a to ( S )- 8a with eight E. coli strains (10 g cdw l −1 ), each containing enzyme module 1, 2 and 4, respectively. ( f ) Time course of biotransformation of 60 mM 1a to ( S )- 8a with E. coli (A-M1_R-M2_C-M4) cells (15 g cdw l −1 ) in a two-liquid-phase system (KP buffer containing 0.5% glucose and 100 mM NH 3 /NH 4 Cl and n -hexadecane; 1:1) at 30 °C (arrow: adding additional 0.5% glucose and 100 mM NH 3 /NH 4 Cl at 20 h). All biotransformations were performed in triplicate, and error bars show±s.d. Full size image Engineering of catalyst to convert alkene to amino alcohol Module 1 and module 3 were combined for the asymmetric aminohydroxylation of alkenes ( Fig. 2b ). Combinatorial assembly of module 1 plasmids (A-M1, C-M1, E-M1 and R-M1) and module 3 plasmids (A-M3, C-M3, E-M3 and R-M3) led to 12 different E. coli strains ( Table 1 ), each co-expressing SMO, SpEH, AlkJ, CvωTA and AlaDH. Biotransformation of 50 mM 1a was examined with resting cells of each E. coli strain in a two-liquid-phase system for 10 h ( Fig. 4c ). All strains produced ( S )- 6a (1–28 mM), and three of them produced ( S )- 6a in 26–28 mM. The best one, E. coli (A-M1_E-M3), gave 28 mM ( S )- 6a (56% conversion) with the accumulation of ( S )- 3a (2 mM), ( S )- 4a (2 mM) and ( S )- 5a (5 mM). The reaction buffer and temperature were then optimized to improve the final product yield ( Supplementary Fig. 8 ). E. coli (A-M1_E-M3) was chosen as the catalyst for this type of biotransformations. The specific activities of E. coli (A-M1_E-M3) towards 1a , ( S )- 2a , ( S )- 3a and ( S )- 4a were 45, 280, 39 and 11 U (g cdw) –1 , respectively. The biotransformation was examined with styrene 1a at 50–80 mM, and 60 mM substrate was found to give the highest concentration of ( S )- 6a ( Supplementary Fig. 7b ). Figure 4d depicted the time curve of the reaction of 60 mM 1a with 15 g cdw l –1 resting cells: 42 mM (5.8 g l –1 ) ( S )- 6a was produced in 98% e.e. and 70% conversion in 12 h. Unreacted substrate 1a , intermediates ( S )- 3a and ( S )- 4a , and by-product ( S )- 5a remained at low concentrations (0.2, 2, 0.1 and 4 mM, respectively). The cascade biocatalysis did not produce phenylglycinol, suggesting the excellent regioselectivity of the aminohydroxylation. Engineering of catalyst to convert alkene to α-amino acid Modules 1, 2 and 4 were assembled together as the catalyst ( Fig. 2c ). Instead of combinatorial assembly of the basic modules, module 4 on four different plasmids (A-M4, C-M4, E-M4 and R-M4) was transformed into the existing best four recombinant E. coli strains containing module 1 and 2, E. coli (A-M1_E-M2), E. coli (A-M1_R-M2), E. coli (C-M1_E-M2) and E. coli (R-M1_E-M2). This generated eight different E. coli strains, each containing module 1, 2 and 4 on different plasmids ( Table 1 ). The eight strains were individually examined for biotransformation of 50 mM styrene 1a to ( S )-phenylglycine 8a ( Fig. 4e ). All strains produced ( S )- 8a (15–40 mM), and five of them produced 37–40 mM ( S )- 8a . E. coli (A-M1_R-M2_C-M4) showed the highest productivity, generating 40 mM ( S )- 8a (80% conversion) in 24 h together with ( S )- 3a , ( S )- 5a and 7a (1 mM each). This strain was chosen for this type of biotransformations. The specific activities of E. coli (A-M1_R-M2_C-M4) towards 1a , ( S )- 2a , ( S )- 3a , ( S )- 4a , ( S )- 5a and 7a , were determined to be 20, 75, 11, 16, 10 and 16 U (g cdw) –1 , respectively. Biotransformations of 50–80 mM 1a to ( S )- 8a were examined, and 60 mM 1a was found to give the highest final product concentration ( Supplementary Fig. 7c ). As shown in Fig. 4f , biotransformation of 60 mM 1a with 15 g cdw l –1 resting cells gave 33 mM ( S )- 8a at 20 h, together with 8 mM 1a and 16 mM 7a . By the additional feeding of 0.5% glucose and 100 mM NH 3 /NH 4 Cl at 20 h, enantiopure ( S )- 8a was produced in 48 mM (7.3 g l –1 ) and 80% conversion at 24 h, with intermediates ( S )- 3a , ( S )- 5a and 7a at low concentrations (3, 0.5 and 1 mM, respectively). Bioconversion of alkenes 1a – k to ( S )-α-hydroxy acids 5a – k To explore the substrate scope and synthetic potential of the asymmetric functionalization of alkenes to α-hydroxy acids, styrenes 1a–k (20 mM) were biotransformed with resting cells of E. coli (A-M1_R-M2) (10 g cdw l –1 ) for 12 h in a two-liquid-phase system (KP buffer and n -hexadecane; 1:1) ( Table 2 ). Five ( S )-α-hydroxy acids ( 5a–d and 5k ) were produced in 90–99% conversion, and six ( S )-α-hydroxy acids ( 5e–j ) were produced in 69–86% conversion. The ( S )-configurations of 5a–k were established by comparing the bioproducts with the commercially available enantiopure standards ( 5a , 5d – f and 5j ) or derived from the previously established ( S )-configurations of the diol intermediates ( 3b , 3c , 3g – i and 3k ) [39] . Ten chiral α-hydroxy acids ( 5a–i and 5k ) were produced in 98–99% e.e., and 5j was obtained in 96% e.e.. The high product e.e. values were generated by the highly enantioselective epoxidation of 1a–k with SMO, regioselective hydrolysis of ( S )- 2a–k with SpEH, and S -selective oxidation of 3a–k with AlkJ. Table 2 Regio- and enantioselective functionalization of terminal alkenes 1a–k to α-hydroxy acids 5a–k with E. coli (A-M1_R-M2) via cascade biocatalysis. Full size table Bioconversion of alkenes 1 a–k to ( S )-amino alcohols 6a–k The substrate scope and synthetic potential of the aminohydroxylation of alkenes were explored with E. coli (A-M1_E-M3) (10 g cdw L −1 ) to transform styrenes 1a–k (20 mM) in a two-liquid-phase system (NaP buffer and n -hexadecane; 1:1) ( Table 3 ). Good conversion (65–86%) was achieved for ( S )-amino alcohols 6a–d and 6i–k in 24 h, while ( S )- 6e–h were produced in relatively low conversion (16–36%). ( S )-configuration of 6a was established by comparing the bioproduct with commercially available enantiopure standard, while ( S )-configurations of 6b–k were derived from the previously established ( S )-configurations of diol intermediates 3b–k [39] . Seven ( S )-amino alcohols ( 6a–b , 6e–g , 6i and 6k ) were produced in 98–99% e.e., three ( S )-amino alcohols ( 6c , 6h and 6j ) were formed in 96–97% e.e. and ( S )- 6d was obtained in 91% e.e.. The high e.e. values were mainly generated by the high enantioselectivity of biotransformation with enzyme module 1. Table 3 Regio- and enantioselective functionalization of terminal alkenes 1a–k to 1,2-amino alcohols 6a–k with E. coli (A-M1_E-M3) via cascade biocatalysis. Full size table Bioconversion of alkenes 1a–k to ( S )-α-amino acids 8a–k The substrate scope and synthetic potential of the asymmetric functionalization of alkenes to ( S )-α-amino acids were examined with resting cells of E. coli (A-M1_R-M2_C-M4) (10 g cdw l –1 ) to convert styrenes 1a–k (20 or 5 mM) in a two-liquid-phase system (KP buffer and n -hexadecane; 1:1) for 24 h ( Table 4 ). ( S )- 8a and ( S )- 8c were produced in excellent conversion of 88 and 91%, respectively. ( S )- 8b and ( S )- 8h were produced in moderate conversion of 55 and 28%, respectively. Seven other ( S )-α-amino acids ( 8d–g and 8i–k ) were produced in good conversion of 60–76%. ( S )-configuration of 8a was established by comparing the bioproduct with the commercially available enantiopure standard, while ( S )-configurations of 8b–k were deduced from the L -selectivity of EcαTA on substrates 7b–k . Remarkably, all produced ( S )-α-amino acids 8a–k were in enantiopure forms (e.e. ≥99%). These very high e.e. values were generated by the highly enantioselective transamination of prochiral α-keto acids 7a–k with EcαTA. Table 4 Regio- and enantioselective functionalization of terminal alkenes 1a–k to α-amino acids 8a–k with E. coli (A-M1_R-M2_C-M4) via cascade biocatalysis. Full size table Preparative biotransformations The synthetic application of the three new types of asymmetric functionalizations of alkenes was demonstrated by the preparative biotransformations to produce two ( S )-α-hydroxy acids, two ( S )-amino alcohols and two ( S )-α-amino acids. The ratio of aqueous buffer and n -hexadecane of the two-phase system was examined for the biotransformations, and 1–5:1 ratios gave similar high conversion for all three types of reactions ( Supplementary Fig. 9 ). Thus, the preparative biotransformations were performed at 5:1 ratio of aqueous buffer: n -hexadecane to reduce the use of organic solvent. Biotransformations of alkenes 1a (100 mM) and 1d (50 mM) with resting cells of E. coli (A-M1_R-M2) (20 g cdw l –1 ) gave ( S )-α-hydroxy acids 5a and 5d in 83 and 80% conversion at 24 h, respectively. Simple extraction and crystallization gave ( S )- 5a (98% e.e.) and ( S )- 5d (98% e.e.) in 72 and 61% yield, respectively. Similarly, biotransformations of alkenes 1a (50 mM) and 1i (25 mM) with resting cells of E. coli (A-M1_E-M3) (20 g cdw l –1 ) afforded ( S )-amino alcohols 6a and 6i in 71 and 63% conversion at 24 h, respectively. Extraction and flash chromatography afforded ( S )- 6a (98% e.e.) and ( S )- 6i (98% e.e.) in 62% and 55% yield, respectively. Finally, biotransformations of alkenes 1a (50 mM) and 1d (25 mM) were carried out with resting cells of E. coli (A-M1_R-M2_C-M4) (20 g cdw l –1 ) for 24 h to give ( S )-α-amino acids 8a and 8d in 81 and 79% conversion, respectively. Simple extraction and evaporation afforded enantiopure ( S )- 8a and ( S )- 8d in 70 and 59% yield, respectively. Cascade biocatalysis is of great importance in green synthesis of chemicals, since it could avoid the waste-generating, time-consuming, and costly separation and purification of intermediates in traditional multi-step process. However, efficient non-natural cascades with more than four enzymatic reactions are rare, and their development is challenging. The modularization concept reported here provides a useful tool for the engineering of complex cascade biocatalysis, which is different from the modularization in synthetic biology to build complex genetic circuits [55] and in metabolic engineering to optimize production of certain metabolites [56] , [57] . In the modular cascade biocatalysis, the appropriate basic modules are designed and engineered to ideally give full conversion with no accumulation of the intermediates. In these aspects, modules 1, 2 and 4 are excellent: they produced 90–98% of the final products in high e.e. from the starting materials, with no accumulation of the intermediates ( Fig. 3a,b,d ). These results were achieved by using enzymes having relatively high activities and using the second enzyme with much higher activity than the first enzyme (SpEH versus SMO; EcALDH versus AlkJ; EcαTA versus HMO) in the module ( Supplementary Table 3 ). In module 3, the conversion of the starting material to the final product reached 70%. Overall, 10% of the intermediate remained, which is possibly due to the relatively low activity of CvωTA for the second reaction, the transamination ( Fig. 3c ). Further improvement of module 3 might be achieved by using other enzymes with higher amination activity. Efficient cascade catalysis systems consisting of multiple basic modules were developed by the combinatorial assembly of the basic modules on different plasmids to adjust the expression level of the enzymes. This method led to the development of E. coli (A-M1_R-M2), E. coli (A-M1_E-M3) and E. coli (A-M1_R-M2_C-M4) as powerful catalysts for the asymmetric functionalizations of alkenes to ( S )-α-hydroxy acids, ( S )-1,2-amino alcohols and ( S )-α-amino acids, respectively. These catalysts enabled the biotransformation of 120 mM 1a to ( S )- 5a in 78% conversion, 60 mM 1a to ( S )- 6a in 70% conversion and 60 mM 1a to ( S )- 8a in 80% conversion, respectively, with low accumulation of the intermediates ( Fig. 4b,d,f ). Since some oxidoreductases were used in the cascade biocatalysis, cofactor recycling has to be considered for efficient biotransformations. While SMO [47] and AlaDH [52] are nicotinamide adenine dinucleotide (NADH)-dependent, GluDH is nicotinamide adenine dinucleotide phosphate (NADPH)-dependent and EcALDH is NAD + -dependent [50] . On the other hand, SpEH [48] , HMO [54] , EcαTA, CAT and CvωTA [51] are independent of nicotinamide cofactors, and AlkJ is a non-canonical ADH coupling to the bacterial respiratory chain instead of nicotinamide cofactors [49] . Therefore, there is no net consumption of the nicotinamide cofactor in the functionalization of styrenes to ( S )-hydroxy acids ( Fig. 2a ). However, 2 moles NADH are needed for producing 1 mole ( S )-amino alcohol from styrene ( Fig. 2b ), and 1 mole NADPH is required for producing 1 mole ( S )-amino acid from styrene ( Fig. 2c ). For these two types of biotransformations with whole-cell biocatalysts, the regeneration of NAD(P)H was achieved via cell metabolism of glucose. This was clearly demonstrated in Fig. 4f : feeding of additional glucose at 20 h significantly improved the conversion of the final product ( S )- 8a . Future improvement of these reactions might be achieved by co-expressing a NAD(P)H-regenerating enzyme in the recombinant biocatalysts. An important parameter in catalysis is the total turnover number (TTN). We calculated the TTN of individual enzymes in the biotransformations based on the amount of the enzymes inside three whole-cell biocatalysts estimated by separation and analysis of the proteins with SDS–PAGE and densitometer ( Supplementary Fig. 10 ; Supplementary Table 4 ). SMO(StyA), SpEH, AlkJ and EcALDH were expressed in E. coli (A-M1_R-M2) at 10, 6.0, 23 and 14 mg protein (g cdw) –1 , respectively, and gave a TTN of 32,000, 51,000, 18,000 and 25,000, respectively, in the biotransformation of 1a to ( S )- 5a ( Fig. 4b ). SMO(StyA), SpEH, AlkJ and CvωTA were expressed in E. coli (A-M1_E-M3) at 13, 6.2, 15 and 7 mg protein (g cdw) –1 , respectively, and afforded a TTN of 13,000, 24,000, 13,000 and 21,000, respectively, in the biotransformation of 1a to ( S )- 6a ( Fig. 4d ). SMO(StyA), SpEH, AlkJ, EcALDH and EcαTA were expressed in E. coli (A-M1_R-M2_C-M4) at 2.8, 1.6, 7.8, 4.6 and 4.6 mg protein (g cdw) –1 , respectively, and gave a TTN of 58,000, 95,000, 26,000, 38,000 and 24,000, respectively, in the biotransformation of 1a to ( S )- 8a ( Fig. 4f ). The good TTN values of these key enzymes indicate the high efficiency of their catalysis in the cascade biotransformations. On the basis of the specific activities of the three whole-cell biocatalysts towards substrate 1a and the corresponding intermediates ( Supplementary Table 5 ), the following bottlenecks could be deduced: alkJ-catalysed oxidation of ( S )- 3a in the transformation of 1a to ( S )- 5a ; CvωTA-catalysed transamination of ( S )- 4a in the conversion of 1a to ( S )- 6a ; and alkJ-catalysed oxidation of ( S )- 3a and HMO-catalysed oxidation of ( S )- 5a in the transformation of 1a to ( S )- 8a . These bottlenecks were also confirmed by some accumulation of ( S )- 3a ( Fig. 4b ), (S)- 5a ( Fig. 4d , possibly due to the oxidation of ( S )- 4a to ( S )- 5a by other enzymes inside the E.coli cells), and both ( S )- 3a and ( S )- 5a at early reaction stage ( Fig. 4f ) in the corresponding biotransformations. On the basis of the determined specific activities of AlkJ, EcALDH, CvωTA and EcαTA (0.19, 1.1, 0.22 and 14 U (mg protein) −1 , respectively) ( Supplementary Table 3 ; Supplementary Fig. 11 ) and the reported specific activities of SMO [58] , SpEH [48] and HMO [59] (2.1, 16 and 1.8 U (mg protein) –1 , respectively), AlkJ and CvωTA are not very active. Since their expression in the whole-cell catalysts is not low, these two enzymes might be replaced with more active enzymes selected from natural sources or enzyme engineering [60] , [61] , [62] to improve the efficiency of the cascade catalysis. On the other hand, HMO has a relatively high activity, but its expression level is low (too low to be estimated). Thus, future improvement might focus on the enhancement of the expression of HMO or replacement of HMO by other enzymes with higher activity and easier expression. In general, the expression of all involved enzymes might be fine-tuned to a high and balanced level by altering other genetic elements, such as promoters and ribosome-binding sites. The engineered whole-cell biocatalysts accept a group of styrene derivatives as substrates for the three types of asymmetric alkene functionalizations. E. coli (A-M1_R-M2) catalysed the biotransformations of eleven alkenes ( 1a–k) to produce the corresponding ( S )-α-hydroxy acids ( 5a–k ) in good conversion (90–99% for five products and 69–86% for six products) and high e.e. (98–99% for ten products and 96% for one product). Biotransformation of the same eleven alkenes ( 1a–k ) with E. coli (A-M1_E-M3) gave the corresponding ( S )-1,2-amino alcohols ( 6a–k ) in high e.e. (96–99% for ten products and 91% for one product) with good conversion (65–86%) for seven products ( 6a–d and 6i–k ) and low conversion (16–36%) for four products ( 6e–h ). E. coli (A-M1_R-M2_C-M4) catalysed the reaction of alkenes 1a–k to produce ( S )-α-amino acids 8a–k in enantiopure form (all ≥99%e.e) with good conversion (88–91% for two products and 55–76% for eight products) except ( S )- 8h (28%). The regio- and enantioselectivity of three types of alkene functionalizations are outstanding. For the low-conversion biotransformations of 1e–h to ( S )- 6e–h and of 1h to ( S )- 8h , 42–63% of unreacted alkenes remained in the reaction mixture. Thus, the SMO-catalysed epoxidation is the main bottleneck in these reactions, which was possibly caused by (a) the relatively low epoxidation activity of SMO towards those styrenes containing a bulky or electron-withdrawing group, (b) the relatively low expression of SMO in E. coli (A-M1_E-M3) and E. coli (A-M1_R-M2_C-M4) and (c) the inefficient cofactor supply and regeneration in the biotransformations. The improvement of these bioconversions might be achieved by enhancing the expression of SMO, co-expressing a NADH-regenerating enzyme, and/or using an engineered SMO with higher activity towards the alkene substrates. The synthetic application of the developed whole-cell biocatalysts and three new types of asymmetric functionalizations of alkenes were clearly demonstrated in the preparation of two ( S )-hydroxy acids, two ( S )-amino alcohols and two ( S )-amino acids. Biotransformations, workup and purification are straightforward, affording 208–1,095 mg (55–72% yield) of ( S )- 5a , ( S )- 5d , ( S )- 6a , ( S )- 6i , ( S )- 8a and ( S )- 8d in 98–99% e.e. The biocatalytic syntheses utilize non-toxic and biodegradable catalysts, consume inexpensive and green stoichiometric reagents (O 2 , NH 3 or glucose) and operate under mild reaction conditions (25–30 °C, atmosphere pressure, etc), thus being greener than many chemical synthetic methods. From organic synthesis perspective, the one-pot asymmetric functionalization of alkenes to give chiral α-hydroxy acids is unique and advantageous over the traditional multi-step synthesis involving many isolation and purification steps. The biocatalytic synthesis is greener and safer than the cyanide-based synthesis using cyanohydrin [43] . It gives high product yield and e.e. from the low-cost alkenes, being more attractive than the reported kinetic resolution (maximum yield: 50%) and asymmetric reduction of α-keto acids (substrates are not cheap) [63] . The one-pot asymmetric functionalization of alkenes to give chiral α-amino acids has also no chemical counterpart and is greener and safer than the cyanide-based Strecker synthesis of chiral α-amino acids [44] . It enables high product yield and e.e. from inexpensive alkenes, being advantageous over the kinetic resolution (maximum yield: 50%) and asymmetric hydrogenation (substrates are not cheap) appoaches [42] . The one-pot conversion of alkenes to chiral 1,2-amino alcohols is a new type of biotransformation and offers an alternative or even better method in some cases to the existing chemical asymmetric aminohydroxylation (oxyamination) [3] , [45] . The biocatalytic aminohydroxylation produces primary amines of the amino alcohols by utilizing ammonia as the nitrogen source, while chemical aminohydroxylation has difficulty in using ammonia. It could also provide much better regio- and enantioselectivity than the chemical methods. As an example for comparison, biotransformation of styrene 1a afforded ( S )-phenylethanolamine 6a in 98% e.e. with 100% regioselectivity, while Sharpless asymmetric aminohydroxylation of styrene 1a gave ( R )-phenylethanolamine (as 4-toluenesulfonyl derivative) in 55% e.e. together with ( S )-phenylglycinol (as 4-toluenesulfonyl derivative) [64] . From biochemical point of view, our synthetic routes from terminal alkenes to chiral α-hydroxy acids, 1,2-amino alcohols and α-amino acids are three novel non-natural pathways containing four to eight reactions, which are unambiguously distinguished from the natural aromatic or aliphatic alkene degradation pathways reported so far [47] , [65] . Nevertheless, the three synthetic pathways were successfully engineered in microbial cells by modular approach and catalysed well the desired non-natural reactions. In comparison with in vitro cascade biocatalysis, the whole-cell approach with a single recombinant strain enables the easy production of the multiple enzymes and the cost-effective biotransformation. This approach opens new possibility of engineering cells for one-pot multi-step biotransformations to manufacture different types of chemicals in a green, selective and cost-effective manner. In summary, we successfully developed three new types of one-pot asymmetric oxy- and amino-functionalizations of terminal alkenes by cascade biocatalysis, simple and green syntheses of a group of useful and valuable ( S )-α-hydroxy acids, ( S )-1,2-amino alcohols and ( S )-α-amino acids in high e.e. and high yields, and a modular approach for engineering efficient one-pot cascade biocatalysis containing more than four concurrent enzymatic reactions. General procedure to engineer recombinant E. coli strains E. coli T7 expression strain (an E. coli B strain derivative) was purchased from New England Biolabs (#C2566I) and used as host strain for all molecular cloning and biocatalysis experiments. The gene module 1 comprising of styA , styB and spEH was constructed previously [39] . AlkJ gene was amplified from the OCT megaplasmid extracted from P. putida GPo1 as reported [49] . Genes of padA , ilvE , gdhA and katE were amplified from the genomic DNA extracted from E. coli K12 MG 1655 with genomic DNA Purification Kit (Thermo Scientific). Ald gene was amplified from the genomic DNA extracted from B. subtilis str.168 with genomic DNA Purification Kit. Codon-optimized cv_2025 gene was synthesized from Genscript based on the sequence from C. violaceum DSM30191 (ref. 51 ). Codon-optimized sco3228 gene was synthesized from Genscript based on the sequence from S. coelicolor A3(2) [54] (see Supplementary Methods for codon-optimized sequences). All genetic constructions were carried out by using standard molecular biology techniques with Phusion DNA polymerase, FastDigest restriction enzymes and T4 DNA ligase (all from Thermo Scientific). PCR primers were synthesized from Integrated DNA Technologies (see Supplementary Table 6 for a full list of key primers). Purification of DNA after electrophoresis or enzyme digestion was performed with E.Z.N.A. Gel Extraction Kit (Omega Biotek), and extraction of plasmids was performed with Axyprep Plasmid Miniprep Kit (Axygen). Basic gene modules 1–4 were constructed on a set of compatible plasmids pACYCDuet-1, pCDFDuet-1, pETDuet-1 and pRSFDuet-1 (Novagen) as individual artificial operon under control of a T7 promoter with one ribosome-binding site before every gene (see Supplementary Methods for details and Supplementary Fig. 12 for enzyme expression). Gene modules were transformed into E. coli T7 competent cells to obtain the E. coli with individual basic modules. Further transformation of other basic genetic module(s) into a constructed E. coli strain containing one or two basic modules gave an E. coli strain containing two or three basic modules for the desired asymmetric alkene functionalizations (see Supplementary Methods for details and Supplementary Fig. 10 for enzyme expression). General procedure to grow E. coli strains Recombinant E. coli strain was first inoculated in 1 ml LB medium containing appropriate antibiotics (50 mg l –1 chloramphenicol, 50 mg l –1 streptomycin, 100 mg l –1 ampicillin, 50 mg l –1 kanamycin or a combination of them) at 37 °C for 7–10 h. The culture was then transferred into 25 ml M9 medium containing glucose (20 g l –1 ), yeast extract (6 g l –1 ) and appropriate antibiotics in a 125 ml tri-baffled flask. The cells were grown at 37 °C and 300 r.p.m. for about 2 h to reach an OD 600 of 0.6, followed by the addition of IPTG to 0.5 mM to induce the enzyme expression. The cells were grown for 12–13 h at 22 °C to reach late exponential phase, and they were collected by centrifugation (3,500 g , 10 min). The cell pellets were resuspended in an appropriate buffer to the desired density as resting cells for biotransformation. General procedure to convert 1a–k to ( S )- 5a–k Overall, 2 ml suspension (10 g cdw l –1 ) of the freshly prepared E. coli (A-M1_R-M2) cells in KP buffer (200 mM, pH 8.0) containing glucose (0.5%, w/v) were mixed with 2 ml n -hexadecane containing one of alkene substrates 1a–k (20 mM). The mixture was shaken at 300 r.p.m. and 30 °C for 12 h, and 150 μl aliquots of each phase were taken out at different time points for following the reaction. For organic phase, 100 μl n -hexadecane were separated after centrifugation (13,000 g , 2 min), diluted with 900 μl n- hexane (containing 2 mM benzyl alcohol as internal standard) and analysed by normal phase HPLC for quantifying alkenes 1a–k and possible epoxides 2a–k . For aqueous phase, 100 μl supernatant were separated after centrifugation (13,000 g , 2 min), diluted with 400 μl TFA solution (0.5%) and 500 μl acetonitrile (containing 2 mM benzyl alcohol as internal standard) and then analysed by reverse phase HPLC for quantifying hydrophilic products 3a–k , 4a–k and 5a–k . To determine the e.e. of 5a–k , the remaining aqueous phase at the end of reaction was separated after centrifugation (13,000 g , 2 min), acidified with TFA and saturated with NaCl, followed by extraction with ethyl acetate and dry over Na 2 SO 4 . After evaporation of ethyl acetate, the residue was dissolved in solvent ( n -hexane: IPA=9:1) for chiral HPLC analysis (see Supplementary Table 7 ; Supplementary Figs 19–29 ; Supplementary Methods for analytic methods). General procedure to convert 1a–k to ( S )- 6a–k Overall, 2 ml suspension (10 g cdw l –1 ) of freshly prepared E. coli (A-M1_E-M3) cells in NaP (sodium phosphate) buffer (200 mM, pH 8.0) containing glucose (1%, w/v) and NH 3 /NH 4 Cl (200 mM, NH 3 :NH 4 Cl=1:10) were mixed with 2 ml n -hexadecane containing one of the alkene substrates 1a–k (20 mM). The mixture was shaken at 300 r.p.m. and 25 °C for 24 h. At 12 h, additional glucose (0.5%, w/v) and NH 3 /NH 4 Cl (100 mM) were added. Samples were taken at different time points and prepared for analysis according to the same procedure described above in the conversion of 1a–k to 5a–k . Alkenes 1a–k and possible epoxides 2a–k were analysed by normal phase HPLC, and hydrophilic products 3a–k , 4a–k , 5a–k and 6a–k were determined by reverse phase HPLC. To determine the e.e. of 6a–k , the remaining aqueous phase at the end of reaction was separated after centrifugation (13,000 g , 2 min), acidified with TFA, and 100 μl sample were separated and diluted with 900 μl TFA solution (0.1%) for chiral HPLC analysis (see Supplementary Table 7 ; Supplementary Figs 30–40 ; Supplementary Methods for analytic methods). General procedure to convert 1a–k to ( S )- 8a–k Overall, 2 ml suspension (10 g cdw l –1 ) of freshly prepared E. coli (A-M1_R-M2_C-M4) cells in KP buffer (200 mM, pH 8.0) containing glucose (0.5%, w/v) and NH 3 /NH 4 Cl (100 mM, NH 3 :NH 4 Cl=1:10) were mixed with 2 ml n -hexadecane containing one of alkene substrates 1a–k (20 or 5 mM). The reaction mixture was shaken at 300 r.p.m. and 30 °C for 24 h. At 20 h, additional glucose (0.5%, w/v) and NH 3 /NH 4 Cl (100 mM) were added. 300 μl aliquots of the mixture (150 μl of each phase) were taken out at different time points for following the reaction. 150 μl HCl solution (0.8M) were mixed with the 300 μl sample, followed by centrifugation (13,000 g , 2 min) to separate the organic and aqueous phases. The procedures for the preparation of the analytic sample from organic phase and the quantification of alkenes 1a–k and possible epoxides 2a–k by normal phase HPLC are the same as the above mentioned ones for the conversion of 1a–k to 5a–k . For aqueous phase, 200 μl supernatant were diluted with 300 μl TFA solution (0.1%) and 500 μl acetonitrile (containing 2 mM benzyl alcohol as internal standard), and the samples were analysed by reverse phase HPLC for quantifying hydrophilic products 3a–k , 4a–k , 5a–k , 7 a–k and 8a–k . To determine the e.e. of 8a–k , the sample preparation and analysis are the same as those described above for the analysis of the e.e. of 6a–k (see Supplementary Table 7 ; Supplementary Figs 41–51 ; Supplementary Methods for analytic methods). Biotransformation of 1a or 1d to prepare ( S )- 5a or ( S )- 5d Overall, 100 ml suspension of E. coli (A-M1_R-M2) cells (20 g cdw l –1 ) in KP buffer (200 mM, pH 8.0) containing glucose (0.5%, w/v) were mixed with 20 ml n -hexadecane containing 1a (10 mmol, 1,042 mg) or 1d (5 mmol, 611 mg). The reaction mixture was shaken at 300 r.p.m. and 30 °C, and 100 μl aliquots of the aqueous phase were taken out at different time points for reversed phase HPLC analysis to follow the reaction. After 24 h, the reaction mixture was subjected to centrifugation (4,000 g , 15 min) to remove the cells and organic phase. The aqueous phase was collected, saturated with NaCl, adjusted to pH>12 with NaOH (10 M) and washed with ethyl acetate two times (2 × 25 ml) to remove trace n -hexadecane and other organic impurities. The aqueous phase was adjusted to pH<2 with HCl (10 M) and extracted with ethyl acetate (3 × 100 ml). The organic phase was collected and dried over Na 2 SO 4 . After filtration, the organic phase was subjected to evaporation by using a rotary evaporator (Buchi Rotavapor R-215) to remove the solvent. The crude hydroxy acid was purified by crystallization in ethyl acetate through dissolving at 65 °C and slowly cooling down to −20 °C. The crystals were taken by filtration, and the mother liquor was evaporated and subjected to crystallization again. The collected crystals were combined and dried overnight under vacuum. ( S )-2-Hydroxy-2-phenylacetic acid 5a : white crystal; 1,095 mg; yield: 72%; e.e. : 98%; [α] D 20 : +146° ( c 1.0, H 2 O) {literature [66] [α] D 20 : +148.8° ( c 0.5, H 2 O), 99% e.e.}. 1 H NMR (400 MHz, D 2 O): δ =7.40–7.36 (m, 5H), 5.22 (s, 1H) p.p.m. ; 13 C NMR (100 MHz, D 2 O): δ =176.2, 138.0, 129.1, 129.1, 127.1, 127.1, 72.9 p.p.m. ( Supplementary Fig. 13 ). ( S )-2-Hydroxy-2-(4-fluorophenyl)acetic acid 5d : white crystal; 518 mg; yield: 61%; e.e. : 98%; [α] D 20 : +141° ( c 1.0, H 2 O) {literature [67] [α] D 28 : +137.3° ( c 0.5, EtOH), 90% e.e.}. 1 H NMR (400 MHz, D 2 O): δ =7.41–7.37 (m, 2H), 7.12–7.08 ( t , J =8.8 Hz, 2H), 5.22 (s, 1H) p.p.m. ; 13 C NMR (100 MHz, D 2 O): δ =176.1, 163.9 and 161.5 (C–F), 134.0, 129.1, 129.0, 115.8, 115.7, 72.2 p.p.m. ( Supplementary Fig. 14 ). Biotransformation of 1a or 1i to prepare ( S )- 6a or ( S )- 6i Overall, 100 ml suspension of E. coli (A-M1_E-M3) cells (20 g cdw l –1 ) in NaP (sodium phosphate) buffer (200 mM, pH 8.0) containing glucose (1%, w/v) and NH 3 /NH 4 Cl (200 mM, NH 3 :NH 4 Cl=1:10) were mixed with 20 ml n -hexadecane containing 1a (5 mmol, 521 mg) or 1i (2.5 mmol, 295 mg). The reaction mixture was shaken at 300 r.p.m. and 25 °C, and 100 μl aliquots of the aqueous phase were taken out at different time points for reversed phase HPLC analysis to follow the reaction. At 12 h, additional glucose (0.5%, w/v) and NH 3 /NH 4 Cl (100 mM) were added. After 24 h, the reaction mixture was subjected to centrifugation (4,000 g , 15 min) to remove the cells and organic phase. The aqueous phase was collected, saturated with NaCl, adjusted to pH<2 with HCl (10 M), and washed with ethyl acetate (2 × 25 ml) to remove trace n -hexadecane and other organic impurities. The aqueous phase was adjusted to pH>12 with NaOH (10 M), followed by extraction with ethyl acetate (3 × 100 ml). The organic phase was separated and dried over Na 2 SO 4 . After filtration, the organic phase was subjected to evaporation. The crude amino alcohol was purified by flash chromatography on a silica gel column with CH 2 Cl 2 :MeOH:NH 3 (28% aqueous solution) of 100:10:1 as eluent ( R f ≈0.2–0.3 for ( S )- 6a and ( S )- 6i ).The collected fraction containing the product was dried over Na 2 SO 4 . After filtration, the organic solvent was removed by evaporation, and the product was dried overnight under vacuum. ( S )-2-Amino-1-phenylethanol 6a : white solid; 425 mg; yield: 62%; e.e. : 98%; [α] D 20 : +46° ( c 1.0, EtOH) {literature [68] [α] D 20 : +48.6° ( c 2.0, EtOH), 99% e.e.}. 1 H NMR (400 MHz, CDCl 3 ): δ =7.37–7.23 (m, 5H), 4.61 (dd, J 1 =8.0 Hz, J 2 =4.0 Hz, 1H); 2.93–2.77 (m, 2H), 2.36 (br, 3H) p.p.m. ; 13 C NMR (100 MHz, CDCl 3 ): δ =142.5, 128.4, 128.4, 127.5, 125.9, 125.9, 74.3, 49.2 p.p.m. ( Supplementary Fig. 15 ). (S)-2-Amino-1-( m -tolyl)ethanol 6i : light yellow syrup; 208 mg; yield: 55%; e.e. : 98%; [α] D 20 : +41° ( c 1.0, EtOH). 1 H NMR (400 MHz, CDCl 3 ): δ =7.26–7.06 (m, 4H), 4.59 (m, 1H); 2.81 (m, 2H), 2.40 (br, 3H), 2.34 (s, 3H) p.p.m. ; 13 C NMR (100 MHz, CDCl 3 ): δ =142.5, 138.1, 128.3, 128.3, 126.6, 122.9, 74.3, 49.1, 21.4 p.p.m. ( Supplementary Fig. 16 ). Biotransformation of 1a or 1d to prepare ( S )- 8a or ( S )- 8d Overall, 100 ml suspension of E. coli (A-M1_R-M2_C-M4) cells (20 g cdw l –1 ) in KP buffer (200 mM, pH 8.0) containing glucose (0.5%, w/v) and NH 3 /NH 4 Cl (100 mM, NH 3 :NH 4 Cl=1:10) were mixed with 20 ml n -hexadecane containing 1a (5 mmol, 521 mg) or 1d (2.5 mmol, 305 mg). The reaction mixture was shaken at 300 r.p.m. and 30 °C, and 100 μl aliquots of the aqueous phase were taken out at different time points for reversed phase HPLC analysis to follow the reaction. At 12 h, additional glucose (1%, w/v) and NH 3 /NH 4 Cl (200 mM) were added. After 24 h, the reaction mixture was subjected to centrifugation (4,000 g , 15 min) to remove the cells and organic phase. The collected aqueous phase was filtered to further remove solid impurities, followed by washing with ethyl acetate (2 × 25 ml) to remove trace n -hexadecane and other organic impurities. After neutralization to pH=7 with NaOH (10 M), the aqueous solution was concentrated to about 15 ml by evaporation to precipitate the amino acid. The solid was collected by filtration, washed with cold water and EtOH and dried overnight under vacuum. ( S )-2-Amino-2-phenylacetic acid 8a : white solid; 528 mg; yield: 70%; e.e. : 99%; [α] D 20 : +148° ( c 1.0, 1 M HCl) {literature [69] [α] D 23 : +150° ( c 1.0, 1 M HCl), 99% e.e.}. 1 H NMR (400 MHz, D 2 O containing 2% H 2 SO 4 ): δ =7.36–7.30 (m, 5H), 5.04 (s, 1H) p.p.m. ; 13 C NMR (100 MHz, D 2 O containing 2% H 2 SO 4 ): δ =170.7, 131.3, 130.4, 129.7, 129.7, 128.1, 128.1, 56.5 p.p.m. ( Supplementary Fig. 17 ). ( S )-2-Amino-2-(4-fluorophenyl)acetic acid 8d : white solid; 250 mg; yield: 59%; e.e. : 99%; [α] D 20 : +138° ( c 1.0, 1M HCl) {literature [70] [α] D 20 : +141° ( c 1.0, 1M HCl), 99% e.e.}. 1 H NMR (400 MHz, D 2 O containing 2% H 2 SO 4 ): δ =7.34–7.31 (m, 2H), 7.08–7.03 (m, 2H), 5.04 (s, 1H) p.p.m. ; 13 C NMR (100 MHz, D 2 O containing 2% H 2 SO 4 ): δ =170.6, 164.6 & 162.2 (C-F), 130.4, 130.3, 127.4, 127.4, 116.7, 116.4, 55.8 p.p.m. ( Supplementary Fig. 18 ). Chemicals Chemicals used in this study are listed in Supplementary Table 8 . Data availability DNA sequence data that support the findings of this study have been deposited in Genbank with the accession codes (SpEH: KX146840; CvωTA: KX146841; HMO: KX146842) or are available in Genbank with the accession codes (SMO: AF031161; AlkJ: AJ245436; EcALDH: 945933; AlaDH: 936557; EcαTA: 948278; GluDH: 946802; CAT: 946234). All other data supporting the findings of this study are available within the article and its Supplementary Information file. How to cite this article: Wu, S. et al. Highly regio- and enantioselective multiple oxy- and amino-functionalizations of alkenes by modular cascade biocatalysis. Nat. Commun. 7:11917 doi: 10.1038/ncomms11917 (2016).